Chiral spin liquid and emergent anyons in a Kagome lattice Mott insulator Topological phases in frustrated quantum spin systems have fascinated researchers for decades. One of the earliest proposals for such a phase was the chiral spin liquid, a bosonic analogue of the fractional quantum Hall effect, put forward by Kalmeyer and Laughlin in 1987. Elusive for many years, recent times have finally seen this phase realized in various models, which, however, remain somewhat artificial. Here we take an important step towards the goal of finding a chiral spin liquid in nature by examining a physically motivated model for a Mott insulator on the Kagome lattice with broken time-reversal symmetry. We discuss the emergent phase from a network model perspective and present an unambiguous numerical identification and characterization of its universal topological properties, including ground-state degeneracy, edge physics and anyonic bulk excitations, by using a variety of powerful numerical probes, including the entanglement spectrum and modular transformations. The low-energy properties of frustrated quantum spin systems—loosely speaking, systems of interacting spins in which the local energetic constraints cannot all be simultaneously satisfied—have fascinated researchers for many decades. These systems arise in the description of the spin degrees of freedom of Mott insulators, that is, insulating states where the fluctuations of the charge degrees of freedom have been suppressed by interactions, whereas the spin degrees of freedom remain free to form non-trivial quantum phases. Such states are found in many materials, but can also be artificially made in the laboratory using cold atomic gases [1] , [2] . In most situations, the spins collectively order into some pattern that can be described through a local order parameter. A more exciting possibility, coined spin liquid phase [3] , is that the spins do not order into such a local pattern; instead, a more exotic state governed by strong quantum fluctuations emerges. In a famous paper in 1987, Kalmeyer and Laughlin [4] hypothesized a scenario where a chiral topological spin liquid (CSL) is formed. In this elusive phase of matter, the spins form a collective state that can only be described in terms of emergent, non-local topological properties. So far, this behaviour has experimentally only been observed in fractional Quantum Hall systems [5] , [6] . Such topologically ordered liquids [7] are characterized through a number of universal properties ranging from topologically protected gapless edge states [8] , [9] and a ground-state degeneracy that depends on the topology of the sample [7] to exotic excitations that carry fractional charge and satisfy neither fermionic nor bosonic exchange statistics [10] . These anyonic particles [11] can serve as key ingredients in topological quantum computers [12] , making them relevant also for technological applications. In the specific case of the chiral spin liquid as proposed by Kalmeyer and Laughlin, the universal properties of the ground state are captured by the bosonic ν =1/2 Laughlin state [13] , [14] . Probably the most striking property of this state are its semionic bulk excitations: when exchanging two such semions, the wave function describing the collective state of the system acquires a complex phase i , in stark contrast to conventional bosons or fermions, where the factor is 1 and −1, respectively. Equally striking is the emergence of a topologically protected chiral edge state with a universal spectrum at the boundary of the sample. This leads to unidirectional transport along the boundary of the sample, while the bulk remains insulating. The correspondence between edge and bulk physics has been used as a powerful experimental probe into the physics of fractional quantum Hall systems. Finally, the ground-state degeneracy of this state depends on the topology of the underlying manifold; for example, when placed on a torus, two ground states are found. Over the last decades, much research has been devoted to finding realistic spin Hamiltonians that have such a chiral topological phase as their ground state, but to this date, the only known examples are Hamiltonians that are unlikely to be relevant for any material [15] , [16] , [17] , [18] , [19] , [20] , [21] , [22] , [23] . Here we study a simple spin model on the Kagome lattice ( Fig. 1a ) that in an appropriate parameter regime offers an effective description of the low-energy properties of the Hubbard model, which is the minimal relevant model for itinerant interacting electrons, in the presence of time-reversal symmetry breaking. 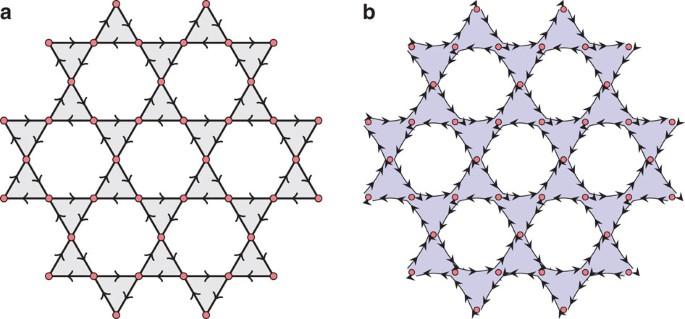Figure 1: Hamiltonian and network model perspective. (a) Kagome lattice considered in this manuscript, where grey shading indicates the elementary triangles. Arrows on the bonds indicate the direction induced by the magnetic flux Φ enclosed in each triangle. (b) Visualization of the network-model perspective on the chiral spin liquid phase arising from Hamiltonian (2). Consistent with a chiral topological phase, a collective edge state encircles the whole systems. In this particular model, additional closed edges encircle each hexagon. The Hubbard Hamiltonian reads Figure 1: Hamiltonian and network model perspective. ( a ) Kagome lattice considered in this manuscript, where grey shading indicates the elementary triangles. Arrows on the bonds indicate the direction induced by the magnetic flux Φ enclosed in each triangle. ( b ) Visualization of the network-model perspective on the chiral spin liquid phase arising from Hamiltonian (2). Consistent with a chiral topological phase, a collective edge state encircles the whole systems. In this particular model, additional closed edges encircle each hexagon. Full size image Here a magnetic field induces both a Zeeman term h z as well as a flux Φ through each elementary triangle of the lattice, such that for i , j , k clockwise around a triangle we have t ij t jk t ki = t 3 exp( i Φ), as indicated by the arrows in Fig. 1a . When Φ≠0 or h z ≠0, time-reversal symmetry is broken. When considered at half-filling, ‹ n ›=1, and in the limit of large repulsive interaction strength U , a Mott insulating state is formed and an effective spin model that captures the low-energy spin physics of the Mott insulator can be derived from perturbation theory in t / U . Here we will demonstrate conclusively that in a very wide parameter regime where a large enough magnetic flux Φ breaks time-reversal symmetry, the ground state of the effective spin model is a CSL with emergent anyonic excitations. It can thus be expected that there is a parameter regime where the full Hubbard model of equation (1) realizes this same phase, but quantitative studies of this question are beyond the current state-of-the-art in numerical techniques and are thus left to future work. Model Starting from the Hubbard model of equation (1), a t / U expansion at half filling gives the following spin Hamiltonian [24] : where for the three-spin term, the i , j , k are ordered clockwise around the elementary triangles of the Kagome lattice. The term , referred to as the scalar spin chirality [25] , [26] , breaks time-reversal symmetry and parity, but preserves SU(2) symmetry. To lowest order, the coupling parameters depend on the parameters of the Hubbard model as J HB ~ t 2 / U and J χ ~Φ t 3 / U 2 , ignoring further subleading terms. We choose to parametrize the model using J HB = J cos θ and J χ = J sin θ and set J =1. In the absence of time-reversal symmetry breaking ( θ =0 and h z =0), this is the Kagome lattice nearest-neighbour Heisenberg antiferromagnet, which has become a paradigmatic model for frustrated magnetism [27] , [28] , [29] with a possible spin liquid ground state and relevance to the description of materials [3] . Recent numerical work [30] , [31] , [32] has indicated that this model may realize a time-reversal symmetric 2 topological spin liquid, whereas other numerical results give evidence for a gapless spin liquid phase [33] , [34] . Here we explore the ground-state phase diagram of equation (2) away from the time-reversal invariant Heisenberg point θ =0. In particular, we find an extended chiral spin liquid phase around the point θ = π /2 and h z =0, where the Hamiltonian reduces to the three-spin term, Our numerical results indicate that the CSL is in fact stable almost up to the Heisenberg point, namely for all θ ≥0.05 π . We also establish an extended range of stability against other perturbations, including the Zeeman field, an easy-axis spin anisotropy in the Heisenberg term, a next-nearest neighbour Heisenberg term, and the Dzyaloshinsky–Moriya interaction [35] , [36] , [37] induced by Rashba-type spin-orbit coupling for the fermions. Although the aim of this paper is not to examine the nature of the transitions out of the chiral spin liquid phase, for example, the expected phase transition to the time-reversal symmetric spin liquid of the Heisenberg antiferromagnet, these questions should be addressed in future work. In the following, we will use two complementary routes to show that the ground state of equation (3) is indeed a chiral spin liquid. First, we argue for this from a powerful perspective rooted in the physics of network models of edge states akin to the Chalker-Coddington network model for the integer quantum Hall transition [38] . We will then turn to powerful numerical tools to unambiguously identify the universal properties of the chiral spin liquid. The key step of our first argument is to view each triangle of spins as the seed of a chiral topological phase, a puddle encircled by an edge state, as illustrated in Fig. 2a . The natural candidate for the phase filling the puddle is the bosonic ν =1/2 Laughlin state [39] , which is the simplest bosonic quantum Hall state known to possess the SU(2) symmetry required by our construction. It is also the state envisioned by Kalmeyer and Laughlin [4] . Forming a lattice out of the elementary triangles, we should then consider a situation with many individual puddles of this topological phase. To see what collective state is formed, we have to understand how two corner-sharing triangles of the Kagome lattice are joined. This situation of edges meeting at the corner spin shared by two triangles is an incarnation of two-channel Kondo physics [40] , [41] , for which it is well-known that the edges will heal [42] , [43] if the coupling to the centre spin is symmetric, as illustrated in Fig. 2b and discussed in more detail in the Methods section. Thus, the corner spin has merged the two triangles to form a larger puddle encircled by a single edge state, that is, to form a larger region of the topological phase. We can repeat the above step ( Fig. 2 ) for all pairs of corner-sharing triangles of the Kagome lattice. The system then forms one macroscopic, extended region of a single topological phase with one edge state encircling its outer boundary, as illustrated in Fig. 1b , and with closed loops encircling the interior hexagons of the Kagome lattice. We thus obtain a direct realization of the Kalmeyer–Laughlin state for a CSL phase. 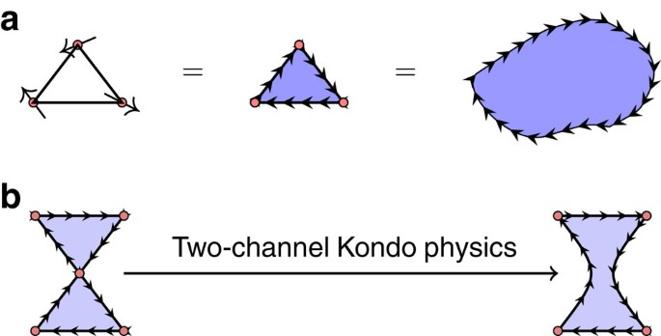Figure 2: Network model perspective. (a) Sketch of a puddle of topological phase replacing each triangle of three spins. (b) Behaviour of two corner-sharing triangular puddles of the topological phase. Figure 2: Network model perspective. ( a ) Sketch of a puddle of topological phase replacing each triangle of three spins. ( b ) Behaviour of two corner-sharing triangular puddles of the topological phase. Full size image Numerical identification of the CSL We now turn to a numerical identification of the CSL at the chiral point θ = π /2 of Hamiltonian (2) and in its vicinity by studying the three hallmark properties of a chiral topological phase: the presence of a gapped spectrum with a topological degeneracy on the torus, a gapless edge state with a universal spectrum of low-energy excitations, and anyonic bulk excitations. On a technical level, we resort to exact diagonalization and density-matrix renormalization group (DMRG) calculations to extract energy spectra, entanglement spectra and modular matrices for various system configurations. To label their diameter and boundary condition, we will use the notation introduced in ref. 30 ; see also the Methods section. We first demonstrate that the system has a finite gap in the thermodynamic limit. To this end, we consider a sequence of XT4-0 tori of length up to 5 unit cells, shown in Fig. 3a . For systems with N ≥18 sites, there clearly is a low-lying excitation, which can be attributed to a twofold near-degeneracy of the ground state. All excitations above these near-degenerate ground states are separated by a spectral gap of roughly Δ≈0.05. Further consistent evidence for the gap can be obtained from exact diagonalization of a 36-site XT6-3 cluster and on XT4-2 clusters of size up to 30 sites (not shown). As a further consistency check, we can extract the gap for long, thin cylinders using DMRG. Performing this for cylinders of type XC4-0 with up to 100 sites, we confirm that the triplet gap does not depend significantly on the length of the system, ruling out the presence of gapless modes propagating along the cylinder. 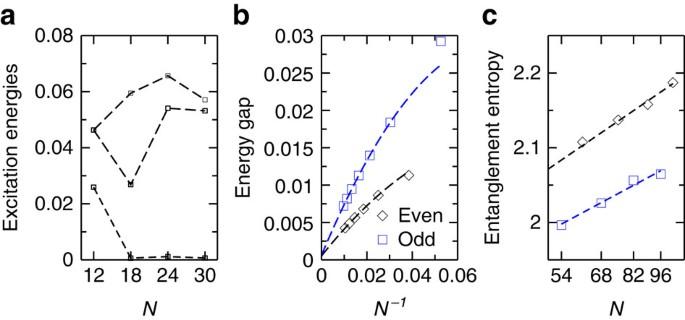Figure 3: Exact diagonalization results. (a) Excitation energies on small tori of type XT4-0 up to length 5. (b) Energy gap on a thin, long strip of width 4 sites; dashed lines indicate the extrapolation toN→∞. The two different branches denote systems with an even (black) and odd (blue) number of unit cells. (c) Entanglement entropy at the centre of the same system as (b) on a semi-logarithmic scale for even (black) and odd (blue) number of unit cells; dashed lines indicate a fit. Both fits are consistent withc=1. In all panels,Nis the total number of lattice sites. Figure 3: Exact diagonalization results. ( a ) Excitation energies on small tori of type XT4-0 up to length 5. ( b ) Energy gap on a thin, long strip of width 4 sites; dashed lines indicate the extrapolation to N →∞. The two different branches denote systems with an even (black) and odd (blue) number of unit cells. ( c ) Entanglement entropy at the centre of the same system as ( b ) on a semi-logarithmic scale for even (black) and odd (blue) number of unit cells; dashed lines indicate a fit. Both fits are consistent with c =1. In all panels, N is the total number of lattice sites. Full size image We conclude from this that the gap remains finite in the thermodynamic limit. The qualitative agreement between the spectral gap extracted for different system sizes and boundary conditions is also a strong indication that the correlation length of the system is short compared with the system sizes we are able to study numerically. To further support this, we have calculated the spin–spin and dimer–dimer correlation functions as well as an upper bound on the asymptotic correlation length on infinite cylinders. All of these indicate a correlation length on the order of one unit cell. Taken together, this gives strong evidence that the properties observed on small tori and quasi-one-dimensional systems are representative of the two-dimensional phase in the thermodynamic limit. The observed twofold near-degeneracy is consistent with what is expected for the CSL, namely a 2 g -fold ground-state degeneracy on a manifold of genus g , which will be split by an amount that is exponentially small in the system size. We also find two states |Ψ a › with very similar energy densities for infinite cylinders of type XC8-4 and XC12-6. As explained in the Methods section, the two states can be identified by their well-defined topological flux a through the cylinder, which for the ν =1/2 Laughlin state can be the identity ( a =) or a semion ( a =s). Edge physics Placing a chiral topological phase on a cylinder or disk, a gapless chiral edge state emerges with a universal spectrum governed by a conformal field theory [8] , [9] . To observe this, we consider the spectral gap of the system when placed on a thin, long strip with a fixed width of four sites. In stark contrast with the case of a thin long cylinder, the spin gap vanishes as a / L + b / L 2 , where a and b are parameters of the fit ( Fig. 3b ). This is a hallmark signature of a gapless edge mode. We can further pinpoint the universality class of the edge theory by extracting its central charge c from the entanglement entropy. As shown in the Fig. 3c , we find good agreement with a value of c =1, which is precisely that expected for the chiral SU(2) 1 Wess–Zumino–Witten conformal field theory describing the edge of a ν =1/2 Laughlin state. As an even more refined probe, we use the entanglement spectrum, which reflects the same universal properties as the physical edge spectrum [44] , [45] , [46] , [47] , [48] . For each of the two ground states |Ψ a › obtained for an infinite cylinder, the entanglement spectrum, see Fig. 4 , is consistent with the corresponding sector of the chiral SU(2) 1 Wess–Zumino–Witten conformal field theory: the entanglement spectrum of |Ψ› displays precisely the sequence of degeneracies of the tower of Kac-Moody descendants of the identity primary field (1-1-2-3-5-...). These are reproduced by counting the number of low-lying close-by states in each tower grouped by momentum and spin quantum numbers. Similarly, the entanglement spectrum of | Ψ s › displays the degeneracies of the spin-1/2 primary field and its descendants (also 1-1-2-3-5-...). We note that in the identity sector, all towers carry integer representations of the spin quantum number, whereas in the semion sector they carry half-integer representations. In both ground states, the levels can be grouped into SU(2) multiplets. 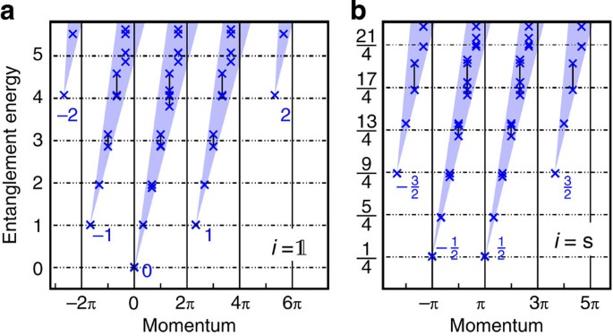Figure 4: Entanglement spectrum. Entanglement spectrum of the reduced density matrixρafor one half of an infinite cylinder obtained for both ground states |Ψ› (a) and |Ψs› (b). The entanglement energies shown on the vertical axis, up to the global shift and rescaling, are given byEa,σ=−log(pa,σ), wherepa,σare the eigenvalues ofρa. The horizontal axis shows the momentum in the transverse direction of the corresponding eigenvectors ofρa. Each tower is identified by itsSzquantum number as indicated by the blue label; we have offset the momentum of different towers by 2πto improve clarity. The cylinder used here is XC12-6, and we show results forθ=0.05π; qualitatively similar results are obtained for all 0.05π≤θ≤0.5π. Figure 4: Entanglement spectrum. Entanglement spectrum of the reduced density matrix ρ a for one half of an infinite cylinder obtained for both ground states |Ψ› ( a ) and |Ψ s › ( b ). The entanglement energies shown on the vertical axis, up to the global shift and rescaling, are given by E a , σ =−log( p a , σ ), where p a , σ are the eigenvalues of ρ a . The horizontal axis shows the momentum in the transverse direction of the corresponding eigenvectors of ρ a . Each tower is identified by its S z quantum number as indicated by the blue label; we have offset the momentum of different towers by 2 π to improve clarity. The cylinder used here is XC12-6, and we show results for θ =0.05 π ; qualitatively similar results are obtained for all 0.05 π ≤ θ ≤0.5 π . Full size image Emergent anyons The bulk of the chiral spin liquid phase has anyonic excitations, referred to as semions. The topological properties of these quasiparticles can be characterized through their modular T and S matrices [12] . The T matrix contains the central charge c and the self-statistics of the anyonic particles, that is, the phase that is obtained when two particles of the same kind are exchanged. The S matrix contains the mutual statistics of the anyonic quasiparticles, their quantum dimensions (counting the internal degrees of freedom of each particle) and the total quantum dimension of the phase. More detailed definitions of these quantities are given in the Methods summary. For a fixed number of quasiparticles, only a finite number of possible S and T matrices exist [49] , [50] . For two types of quasiparticles (as in the case of the ν =1/2 bosonic Laughlin state), only two choices are possible [49] . Therefore, by numerically calculating the S and T matrices and comparing them against the two possibilities, we have fully identified the universal properties of the topological phase. For the ν =1/2 Laughlin state, the modular matrices are For an XT8-4 torus of 48 sites at θ =0.05 π , where the finite-size corrections to this quantity are minimal, we obtain This is in very good agreement with the T and S matrices for the ν =1/2 Laughlin state given in equation (4) and provides the strongest confirmation of the nature of the bulk topological phase. The correct normalization of the first row or column of the S matrix indicates that we have indeed obtained a full set of ground states. We can also read off the total quantum dimension of the phase, which determines the topological entanglement entropy [51] , [52] that has been widely used to identify topological phases. Furthermore, the central charge c =0.988, as obtained from the T matrix, is in excellent agreement with the prediction and the value extracted from the edge above. Stability of the chiral spin liquid phase To establish the region in which the phase persists as θ is tuned in the range θ ε[0, π /2], we first consider the fidelity [53] F ( θ )=‹Ψ a ( θ − ε )|Ψ a ( θ + ε )› shown in Fig. 5 (for the precise definition of this quantity for infinite systems, see the Methods section). The fidelity remains near unity as θ is tuned away from the chiral point θ = π /2, until it suddenly drops for θ <0.05 π , indicating a transition in the regime 0< θ <0.05 π . Further support for the extended stability of the CSL is found in various other characteristics, including the spectral gap, the modular matrices and the entanglement spectrum. This is remarkable as it indicates that tuning away from the Heisenberg model ( θ =0) with a small critical chiral coupling of ( J χ / J HB ) crit ≤tan(0.05 π )≈0.16 is sufficient to drive the system into the chiral phase. We emphasize that this is merely an upper bound for the location of the transition. 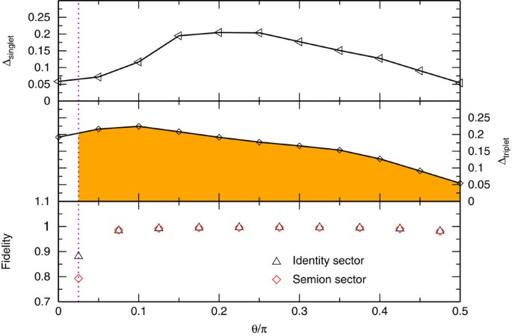Figure 5: Excitation gaps. Singlet and triplet gaps as a function ofθfor an infinite XC8-4 cylinder. The triplet gap is a lower bound on the critical magnetic fieldhc; hence, the shaded region indicates the minimal stability of the phase in theθ-hzphase diagram. Figure 5: Excitation gaps. Singlet and triplet gaps as a function of θ for an infinite XC8-4 cylinder. The triplet gap is a lower bound on the critical magnetic field h c ; hence, the shaded region indicates the minimal stability of the phase in the θ - h z phase diagram. Full size image In experimental scenarios, a Zeeman magnetic field h z is likely to be generated along with the orbital magnetic field that induces the three-spin chiral term. The relative strength of the orbital magnetic field and the Zeeman field is determined by the g -factor and the ratio t / U . The energy gap in the triplet sector gives a lower bound on the critical field strength h c up to which the CSL phase is stable. The values for the triplet gap shown in Fig. 5 remain large all the way from the fully chiral point ( θ = π /2) to the transition out of the CSL towards the Heisenberg point ( θ =0). In Fig. 5 , we also show the singlet gap, that is, the gap to the lowest excitation in the S z =0 sector. As opposed to the triplet gap, which appears to remain large across the transition, the singlet gap decreases as the transition out of the CSL is approached. Note that the gaps may be rounded off at the transition by effects owing to either the finite diameter or the finite bond dimension of the matrix-product state ansatz. We point out, however, that a closing only of the singlet and not the triplet gap would be consistent with the scenario for the transition from the chiral spin liquid into a doubled semion phase (twisted 2 topological phase) studied in ref. 54 . We have taken an important step towards physically motivated models for a chiral spin liquid in a frustrated spin system. We believe that this will nucleate new research efforts both by theorists and experimentalists. From a theoretical point of view, studying the transition from the chiral spin liquid to the putative time-reversal symmetric spin liquid in the Heisenberg model will provide the unique opportunity to study a topological phase transition in a realistic model, and may provide invaluable insights into the physics of frustrated spins on the Kagome lattice. For experimentalists, our work will provide a guide in searching for realizations of bosonic fractional Quantum Hall physics in the laboratory, be it in materials that have Kagome lattice structure and form Mott insulators, or by engineering such systems in cold atomic gases. We have so far left unanswered the question of specific parameters that are required to drive a material into the chiral spin liquid phase. The relevant microscopic parameters are the ratio t / U that controls fluctuations around the Mott insulator, and the orbital magnetic field Φ that drives the chiral three-spin term, see equation (1). The ratio J χ / J HB grows as either t / U or Φ is increased, and is to lowest order linear in both; however, in the relevant regime close to the Mott transition, where the three-spin term is expected to be strongest, corrections to this linear dependence are likely to be important and inferring quantitative conclusions about the relevant parameters in the Hubbard model from our results for the effective spin model is thus challenging. The upper bound on the critical coupling ratio J χ / J HB given above thus should only serve as a guide to more detailed simulations of the original Hubbard model, which will allow for a reliable quantitative estimation of the relevant regime of microscopic parameters t / U and Φ. Finally, the orbital magnetic field that can be attained in the laboratory depends very much on material parameters such as the spacing between magnetic moments, which may be larger than the lattice spacing; giving quantitative estimates along with an analysis of candidate materials thus goes beyond the scope of this manuscript. A more detailed treatment of these questions can be found in the Supplementary Note 2 . Another important question is that of how the chiral spin liquid can be identified reliably in an experiment. The most powerful signature of universal behaviour can be found in the thermal transport properties [55] . Although harder to measure than charge transport, which has been used as the most powerful probe of fractional Quantum Hall physics in two-dimensional electron gases, such thermal transport measurements have recently been performed successfully both on 2 d electron gases as well as candidate spin liquid materials [56] . A charge response should also be present, but will not be universal and thus a less powerful indicator of the chiral topological phase. During completion of this work, we became aware of related work in refs. 57 , 58 . Overview In the following, we give a brief overview of the main methods used in our work. Further technical details will be given further below. We label the system sizes according to the scheme introduced in ref. 30 . For cylinders, the labels are XC m - n ; here, X indicates the orientation of the cylinder, m is the diameter of the cylinder in measured sites and n is the shift of the boundary condition when wrapping the plane to a cylinder. Note that cylinders of type XC(2 n )- n are spanned by the basis vectors of the triangular lattice. For tori, we use the labels XT m - n , where m and n have the same meaning as above. Two examples are shown in Fig. 6 . 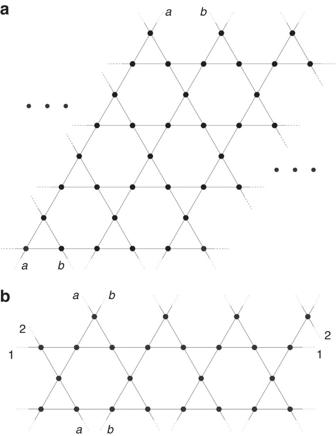Figure 6: Lattices. (a) Section of an XC8-4 cylinder. Links with the same letters/numbers are identified. (b) XT4-0 torus with 24 sites. Figure 6: Lattices. ( a ) Section of an XC8-4 cylinder. Links with the same letters/numbers are identified. ( b ) XT4-0 torus with 24 sites. Full size image We numerically study finite systems using exact diagonalization as well as the DMRG method [59] , [60] . Although our exact diagonalization is limited to 36 sites, DMRG allows us to study systems in a limit of long, thin cylinders and strips. Up to M =4,000 states are used in the finite-size DMRG calculations. Finite-size DMRG calculations allow us to extract the spin gap as well as the entanglement entropies for continuous blocks of sites, which we use to extract the central charge of the system by fitting to the well-known formulas of ref. 61 . Furthermore, we use infinite-size DMRG with a translationally invariant matrix product state ansatz of up to M =4,096 states. This allows us to obtain a complete set of ground states with well-defined anyonic flux, as first proposed in ref. 62 . Here the use of an infinite cylinder (as opposed to a finite cylinder with boundaries, where there is no ground-state degeneracy) is key to obtain one ground state for each anyonic charge, analogous to the torus. In this basis, we can extract the entanglement spectrum as well as the T and S matrices. Reference [62] details the non-trivial step of resolving the entanglement spectrum by transverse momentum. The T and S matrices are defined through a world-line diagram for anyonic particles as (see for example, refs. 12 , 63 ) Here is the total quantum dimension of the phase, and d a is the quantum dimension of a quasi-particle of topological charge a . These matrices can be related to generators of the modular group on the torus, and fulfill the conditions ( ST ) 3 = S 2 and S 4 =1. The T -matrix is proportional to the twist factors Θ a , which contain the self-statistics of the excitations, that is, the phase that is obtained when two particles of the same kind are exchanged once; we have Θ=1. The T matrix has a prefactor e − i (2 π )/(24) c = T , where c is the central charge of the anyon model. The S -matrix contains the mutual statistics, that is, the statistics obtained when particles of general types a , b are braided around each other. The first row of the S matrix contains the quantum dimensions d a of the quasiparticles. To numerically obtain these matrices, first a quasi-orthonormal basis {|Ψ a tor ›} on a torus of 3 × L × L sites with well-defined topological flux a through the torus and a π /3 rotational symmetry must be obtained. As pointed out in ref. 64 , the modular matrices T and S of the emergent anyon model are related to the matrix elements of a π /3 rotation R π /3 through the equation Here D is a diagonal matrix containing only complex phases; it accounts for the freedom in choosing the phases of the vectors |Ψ a tor ›. In ref. 62 , it was shown how to build the basis |Ψ a tor › from an matrix product state (MPS) representation for |Ψ a cyl › and how to extract both T and S from ‹Ψ a tor | R π /3 |Ψ b tor ›. Note that the matrix T is referred to as U in the reference. Finite-size DMRG To study the finite cylinders and strips discussed in the main text that are beyond the system size amenable to exact diagonalization, we use the DMRG method [59] , [60] . Although for many years limited to one-dimensional systems by its exponential scaling in the width of quasi-one-dimensional systems, recent years have seen a surge in applications of large-scale DMRG calculations to 2d systems [65] . A key point is that although it scales exponentially in the width of the system, the scaling is polynomial in the length, allowing it to go much beyond exact diagonalization if boundary conditions and the mapping to a one-dimensional system are chosen appropriately. DMRG is based on a variational ansatz that can be systematically improved by increasing the number M of states kept, where the computational cost grows as ( M 3 ). For the calculations shown in Fig. 3 of the main text, we use up to M =4000 states. From DMRG, we can easily extract the entanglement entropy for a contiguous block of sites at the end of an open system. This allows us to calculate the central charge of a gapless quasi-one-dimensional system by performing a fit to the well-known results of refs. 61 , 66 , which for the entanglement entropy of a contiguous block of n = N /2 sites in an open 1 d system of N sites is Infinite-size DMRG We use infinite-size DMRG to efficiently obtain ground states, parametrized through translationally invariant matrix-product states, on infinite cylinders up to XC12-6 and with up to M =4,096 states, exploiting a U(1) symmetry of the system. The calculation of the entanglement spectrum as well as the modular matrices has been explained in the Methods summary; below, we provide additional detail on numerical parameters used. We also discuss how to extract the fidelity and the bulk gaps from such an infinite ansatz. The approach to extracting the T and S matrices outlined in the Methods summary requires the calculation of the matrix elements of ‹Ψ a tor | R π /3 |Ψ b tor ›, where R π /3 is a 60° rotation. The cost of an exact calculation of this matrix scales as a very large power in the bond dimension M , and in practice, we have to resort to sampling techniques to obtain an approximate evaluation. The results of equation (5) of the main text were obtained using 2 × 10 5 samples over spin configurations in the S z basis using a Markov chain Monte–Carlo update scheme. We have checked that the values for T and S are converged to within 10 −3 . Therefore, the main source of the deviation between the numerically obtained results and the exact matrices is due to finite size effects. Although the calculation of the fidelity is straightforward in the case of finite-size DMRG and exact diagonalization, more care must be taken in the case of infinite-size DMRG as all states are either equal or orthogonal in the thermodynamic limit. In the case of translationally invariant infinite MPS, one can consider the spectrum of the transfer operator of the product of two normalized infinite MPS. Given the eigenvalue with largest absolute value | λ |ε[0,1] of this transfer operator, the overlap of the states for N sites is | λ | N . Clearly, as N →∞, λ N →0 or 1. Therefore, instead of the overlap we quote directly the absolute value of the eigenvalue | λ |, which shows the same behaviour as the fidelity for finite systems. We use ε =0.025. In standard DMRG calculations, the triplet gap is easily available by changing the total spin quantum number of the target state, which is enforced exactly. The singlet gap can be obtained by first converging the ground state of the system and then optimizing a second state under the constraint of orthogonality against the ground state. For infinite-size DMRG calculations, however, neither of these methods are applicable, and we therefore must resort to a different approach. For this manuscript, we choose to approximately extract the gaps from the spectrum of an effective local Hamiltonian obtained by contracting a network of the MPS with the matrix-product operator representation of the Hamiltonian everywhere except on one bond. To validate our approach, we compare the energy gaps extracted from infinite cylinders to small tori of the same diameter. Note that a comparison against finite-size DMRG on long cylinders is hampered by the gapless edge that emerges in that topology. In Fig. 7 , we compare infinite XC4-2 cylinders against an XT4-2 torus with 30 sites, as well as infinite XC8-4 cylinders against an XT6-3 torus with 36 sites. The energies for the tori are mostly obtained with DMRG using up to M =4,000 states; for both sizes, we have performed exact diagonalization calculations at selected values of θ to confirm the ground-state energies obtained from DMRG are within 1% error of the exact energies. The good agreement between the two methods clearly validates the approach used. We have also verified for various values of θ that for XC8-4, the gaps above the two ground states corresponding to different topological sectors are comparable. We therefore only show results for infinite cylinders in the main text. 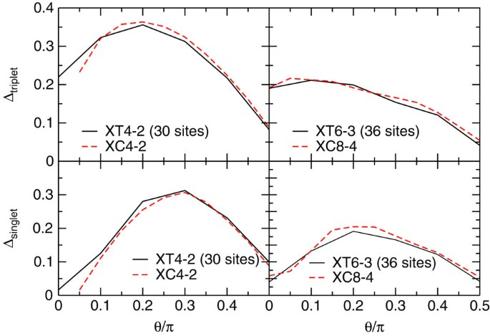Figure 7: Finite- vs infinite-size behaviour of spectral gaps. Comparison of singlet and triplet gaps obtained for infinite cylinders (XC8-4 and XC4-2) as well as for finite tori using DMRG and exact diagonalization of up toN=36 sites. All infinite-size results have been extrapolated to theM→∞ limit. Figure 7: Finite- vs infinite-size behaviour of spectral gaps. Comparison of singlet and triplet gaps obtained for infinite cylinders (XC8-4 and XC4-2) as well as for finite tori using DMRG and exact diagonalization of up to N =36 sites. All infinite-size results have been extrapolated to the M →∞ limit. Full size image Network model We now revisit the network model perspective discussed in the main text, and provide additional detail on how the healing of the edge states surrounding two corner-sharing triangles that share one spin can be understood in terms of two-channel Kondo physics. If we envision the puddles to be very large, they would carry the edge state on each side and the corner would look as shown in Fig. 8Ia . The pair of edge states on the upper triangle is known [10] , [39] to be described by the same theory as the right- and left-movers of a semi-infinite uniform spin-1/2 Heisenberg chain, and analogously for the lower pair of edge states. The spin at the corner then appears as the centre spin of an infinite chain (Fig. 8Ib,Ic). It is well known that the infinite chain will heal if the centre spin is coupled to the two semi-infinite chains with equal strength [42] , [43] . Then, the right- and left-movers will extend throughout the entire, infinite system (Fig. 8Id). The effect on the corner spin is summarized in Fig. 8II , where the situation shown in Fig. 8IIa corresponds to Fig. 8Ia, whereas Fig. 8IId corresponds to Fig. 8Id. As is evident from Fig. 8IId, the corner spin has merged the two triangles to form a larger puddle encircled by a single edge state, that is, to form a larger region of the topological phase. 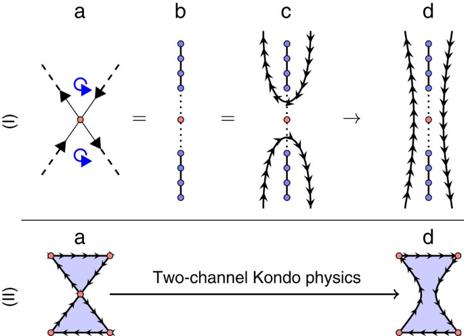Figure 8: Network model construction. (I) Illustration of the behaviour of the edge states at a corner shared by two puddles. (II) Behaviour of two corner-sharing triangular puddles of the topological phase. Figure 8: Network model construction. (I) Illustration of the behaviour of the edge states at a corner shared by two puddles. (II) Behaviour of two corner-sharing triangular puddles of the topological phase. Full size image We can illustrate the validitiy of the above network model picture by considering the different situation where the spins are replaced by Majorana fermion zero modes. The resulting network model will describe a different topological phase. Specifically, replace the spin chirality term on each triangle by a chiral hopping term , which also has the effect of introducing the notion of a chirality on each triangle. This model, which is quadratic in fermionic operators, can be diagonalized straightforwardly. As the Kagome lattice is obtained as a triangular lattice of three-site unit cells, we obtain three energy bands E α ( k x , k y ), α =1,2,3. We observe that all three bands are separated by a gap from each other, and the central band E 2 is dispersionless, that is, E 2 ( k x , k y )=0. Noting that the number of states in this band coincides with the number of hexagons in the system, we identify these zero-energy states as the non-interacting edge states encircling those hexagons of the Kagome lattice (shown in Fig. 1b ) in which a fermion zero mode resides. We calculate the Chern number C (ref. 67 ) using the real-space method of refs. 68 and find that C of the top and bottom band is C =±1, that is, that the model is in a topological phase; this was previously observed in ref. 69 . How to cite this article: Bauer, B. et al. Chiral spin liquid and emergent anyons in a Kagome lattice Mott insulator. Nat. Commun. 5:5137 doi: 10.1038/ncomms6137 (2014).